Global metabolic network reorganization by adaptive mutations allows fast growth ofEscherichia colion glycerol Comparative whole-genome sequencing enables the identification of specific mutations during adaptation of bacteria to new environments and allelic replacement can establish their causality. However, the mechanisms of action are hard to decipher and little has been achieved for epistatic mutations, especially at the metabolic level. Here we show that a strain of Escherichia coli carrying mutations in the rpoC and glpK genes, derived from adaptation in glycerol, uses two distinct metabolic strategies to gain growth advantage. A 27-bp deletion in the rpoC gene first increases metabolic efficiency. Then, a point mutation in the glpK gene promotes growth by improving glycerol utilization but results in increased carbon wasting as overflow metabolism. In a strain carrying both mutations, these contrasting carbon/energy saving and wasting mechanisms work together to give an 89% increase in growth rate. This study provides insight into metabolic reprogramming during adaptive laboratory evolution for fast cellular growth. The genotype–phenotype relationship is fundamental in biology. Adaptive laboratory evolution can now be used to carry out controlled evolutions under defined selection pressures to produce new and fit phenotypes [1] , [2] , [3] , [4] , [5] . Re-sequencing has allowed the detailed assessment of the genetic changes that occur during adaptation [6] , [7] and allelic replacement can be used to ascertain the causality of the observed mutations relative to the observed phenotype [8] . Moreover, next-generation sequencing has made the determination of mutations occurring during adaptation commonplace [9] . However, the genotype–phenotype relationship is multilayered and hierarchical and the measured genotypes and phenotypes are the opposite ends of this hierarchy. The in vitro assessment of the effects of the mutated gene products relative to the wild type (WT) can help determine how molecular properties change [10] , [11] but studies at the level of individual gene-product properties give limited insights into the mechanisms that change the phenotype. Network-level changes resulting from the introduction of causal mutations can now be characterized through the generation and integrative analysis of polyomic data sets. Here we provide a detailed network-level analysis, based on polyomic data sets, of the effects of individual causal mutations found during adaptive laboratory evolution of E. coli . These network-wide measurements are then combined to produce one of the first metabolic studies of two epistatic mutations that improve growth on glycerol. The first whole-genome comparative sequencing study that included allelic replacement of mutations showed that as few as two to three causal mutations can lead to significant changes in growth rate of E. coli during adaptation to glycerol minimum medium [8] . Most of the acquired mutations affecting growth phenotype can be grouped into those affecting condition-specific function (for example, glycerol kinase or glpK ) or global transcription patterns (for example, RNA polymerase β′ subunit encoded by rpoC ). Although the biochemical characteristics of some of the naturally occurring mutations in glycerol kinase and RNA polymerase have been studied [10] , [11] , the underlying molecular and network-level consequences and mechanisms promoting cell growth in vivo have not been uncovered. While adaptive evolution and identification of mutations by re-sequencing has been made easy and cheap, the elucidation of network-level mechanisms remains a major bottleneck in the study of adaptive evolution [4] , [12] . In the current study, we perform comprehensive cellular and exo-metabolome analysis, proteomics, lipidomics and phenotypic characterization of WT and mutant strains of E. coli to investigate the metabolic consequences of two specific adaptive mutations ( glpK 218a>t and rpoC 27 bp deletion) identified in a glycerol-evolved strain. To disentangle the contribution of different mutations, we present data on MG1655 WT and strains harbouring the individual (GLPK and RPOC strains) or combined mutations (DKI strain). The latter’s growth phenotype reconstitutes the glycerol-evolution end point strain (GB) [8] . Our findings provide an overall picture of metabolic network reorganization induced by two adaptive mutations, leading to significant increase in growth rate. Two contrasting strategies that optimize a trade-off between biomass yield by carbon saving and increased carbon flow and metabolic overflow are combined to allow fast growth on glycerol. Globally, these results reveal important metabolic regulatory events under evolutionary selection for fast growth on a non-fermentable carbon source. Glycerol uptake is affected by glpK and rpoC mutations We used 1 H-NMR spectroscopy to monitor change in glycerol concentration in culture medium at different time points during exponential growth over an optical density (OD) 600 of 0.05–0.75 to evaluate the glycerol uptake rate. It took about 10 h for the DKI strains to reach an OD 600 of 0.75, faster than the RPOC (11 h), GLPK (13 h) and WT (16 h) strains. The altered growth rates ( Fig. 1a ) are associated with differences in cell size, as expected, and all data and analysis in this study take cell size into account for normalizing concentrations (see Methods section and Supplementary Fig. 1 ). For all studied strains, we found that less than half of the available glycerol had been consumed at the last sampling point, showing that glycerol was not limiting during the course of the experiment ( Supplementary Fig. 2 ). Compared with the WT strain, glycerol uptake rates for all single- and double-mutant strains were increased by 30–66% ( Fig. 1b ). 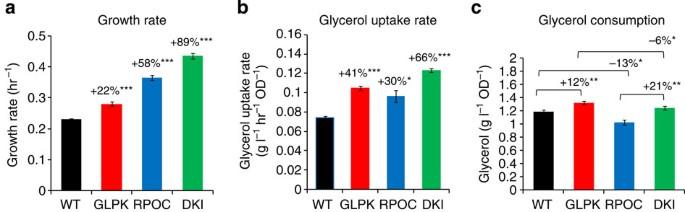Figure 1: Growth-related parameters of WT and mutant strains. (a) Growth rates of the WT and mutant strains on glycerol.Pvalues were obtained using at-test comparing mutants strains with the WT (***P<0.001). (b) Glycerol uptake rate (*P<0.05, ***P<0.001,t-test compared with WT). (c) Glycerol consumption (*P<0.05, **P<0.01, two-group comparison usingt-test). Plots show the mean±s.e. (n=6). Figure 1: Growth-related parameters of WT and mutant strains. ( a ) Growth rates of the WT and mutant strains on glycerol. P values were obtained using a t -test comparing mutants strains with the WT (*** P <0.001). ( b ) Glycerol uptake rate (* P <0.05, *** P <0.001, t -test compared with WT). ( c ) Glycerol consumption (* P <0.05, ** P <0.01, two-group comparison using t -test). Plots show the mean±s.e. ( n =6). Full size image As an index of biomass yield, we monitored the amount of glycerol consumed for each unit of increase in culture optical density for each strain ( Fig. 1c ). Consistent with previous results [11] , biomass yield was increased by the rpoC mutation (expressed as decreased glycerol consumption for equal biomass increase), although it grew faster than both WT and GLPK ( Fig. 1a ). This suggests that strains with this mutation are more efficient in biomass conversion. In contrast, glpK mutation caused increased glycerol consumption for equivalent biomass yield, suggesting that this mutation accelerates growth through increased but less efficient carbon utilization. The rpoC mutation improves metabolic efficiency To elucidate the underlying consequences of adaptive evolution, we performed a combination of metabolomic, lipidomic and proteomic analyses on the strains. For metabolomics, we identified 121 metabolic features present across all samples using capillary electrophoresis mass spectrometry ( Supplementary Fig. 3 and Supplementary Data 1 ). At an OD 600 of 0.25, the concentrations of 68 metabolites were significantly affected by the rpoC mutation ( Fig. 2a , two-way analysis of variance, Bonferroni-corrected P <0.05, n =6), revealing the major changes in the metabolome due to this specific mutation. In addition, 23 metabolite changes were observed as a result of glpK mutation ( Supplementary Fig. 4 ). The large and strain-specific differences in metabolite profiles are also apparent in the results of multivariate analysis (partial least squares discriminant analysis; PLS-DA) of the metabolomic data collected for all strains and sampling points. Strains were clearly separated based on their rpoC genotype in the first PLS-DA component, and based on their glpK genotype in the second PLS-DA component ( Fig. 2b ). 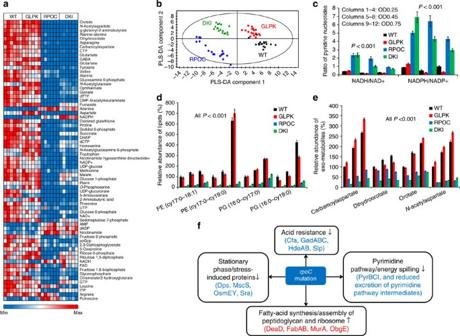Figure 2: Broad metabolic changes associated with therpoCmutation increase metabolic efficiency. (a) Heat map of a subset of 68 identified metabolites examined at OD600of 0.25 (early exponential phase), whose concentrations were significantly affected by therpoCmutation (all Bonferroni-correctedP<0.05). Metabolites are ordered by increasingPvalue from top to bottom (colours indicate min–max normalized relative concentration: blue, minimum concentration; red, maximum concentration). (b) PLS-DA analysis of the global metabolomic data for all 121 metabolites at OD600of 0.25, 0.45 and 0.75 (R2X=0.43, R2Y=0.77,Q2=0.74 for the first three components). (c) Specific changes in NAD(P) metabolite ratios. (d) Specific changes in lipid metabolites and, (e), specific changes in selected exo-metabolites. (f) Summary of main proteomic changes due to therpoCmutation. Plots inc–eshow the mean±s.e. (n=6).Pvalues obtained from two-way analysis of variance (n=18). All values ind,eare calculated relative to levels in WT at OD of 0.25 (100%). Figure 2: Broad metabolic changes associated with the rpoC mutation increase metabolic efficiency. ( a ) Heat map of a subset of 68 identified metabolites examined at OD 600 of 0.25 (early exponential phase), whose concentrations were significantly affected by the rpoC mutation (all Bonferroni-corrected P <0.05). Metabolites are ordered by increasing P value from top to bottom (colours indicate min–max normalized relative concentration: blue, minimum concentration; red, maximum concentration). ( b ) PLS-DA analysis of the global metabolomic data for all 121 metabolites at OD 600 of 0.25, 0.45 and 0.75 (R 2 X=0.43, R 2 Y=0.77, Q 2 =0.74 for the first three components). ( c ) Specific changes in NAD(P) metabolite ratios. ( d ) Specific changes in lipid metabolites and, ( e ), specific changes in selected exo-metabolites. ( f ) Summary of main proteomic changes due to the rpoC mutation. Plots in c – e show the mean±s.e. ( n =6). P values obtained from two-way analysis of variance ( n =18). All values in d , e are calculated relative to levels in WT at OD of 0.25 (100%). Full size image In Fig. 2a , the most striking and global change in the metabolic state is the reduced concentration of most metabolites induced by the rpoC mutation. We ruled out that cell volume effects between strains (dilution) could be responsible for the general decrease in most metabolites (see Methods and Supplementary Fig. 1 ). Notable exceptions include increases in both reduced dinucleotide redox cofactors NADH and NADPH, adenine, dADP, nicotinamide, and putrescine. Most of these changes were also reflected by similar changes in the DKI strain. Ratios of reduced/oxidized metabolites were calculated to better describe redox state and are shown in Fig. 2c ). For WT, the observed reduced/oxidized dinucleotide ratios were comparable to previously reported data for WT on glucose minimal media (NADH/NAD + , 0.31; NADPH/NADP + , 1.05) [1] . However, for both RPOC and DKI strains, the rpoC mutation caused on average a fivefold increase in NADH/NAD + ratio and a sevenfold increase in NADPH/NADP + ratio, as compared with the WT and GLPK strains. The ratios of several other key reporters of redox and nitrogen metabolism are shown in Supplementary Fig. 5 . The large increases in reduced/oxidized dinucleotide ratios following rpoC mutation provide a driver for anabolism, reflected in the lower energy charge while the decrease in glutamine–glutamate/2-ketoglutarate ratios suggest high nitrogen turnover for amino acid/protein production ( Supplementary Fig. 5 ). Consistent with this finding, both RPOC and DKI strains showed increased levels of proteins involved in fatty-acid synthesis (FabAB), and assembly of peptidoglycan (MurA) as well as ribosome biogenesis (ObgE, DeaD; Supplementary Fig. 6 ). Together, these results suggest that the rpoC mutation improves growth through major reorganization of the metabolic network that reflects increased anabolic needs to cope with rapid growth. Moreover, since the growth rate enhancing effects of the rpoC mutation are observable only on minimal media [11] , these global changes can also be interpreted as depicting a response optimizing the synthesis of most biomass precursors, which might explain the generally lower levels of precursor metabolites. To further detail the metabolic effect of adaptive mutations, we performed lipidomic analysis. Consistent with the known major lipid species in E. coli [13] , [14] , [15] , [16] , we observed 22 lipids mainly in the forms of phosphatidylethanolamine and phosphatidylglycerol. Interestingly, the main changes in lipid composition were due the rpoC mutation, as both RPOC and DKI strains showed sharply reduced concentrations in phospholipids that contain cyclopropane fatty acids (CFA) such as cy17:0 and cy19:0 ( Fig. 2d and Supplementary Fig. 7 ). The proteomic data also revealed that the level of CFA synthase (Cfa), the key enzyme for cyclopropanation was reduced sixfold in both RPOC and DKI strains ( Supplementary Fig. 6 ) supporting and explaining the origin of the change in cyclopropane containing lipids. Previous studies have shown that cyclopropanation of fatty acids, a post-synthesis lipid modification, begins normally when the cells enter stationary phase until all unsaturated fatty acids are modified into their corresponding CFA (for example, modification from 16:1 to cy17:0) [17] . The conversion is energetically costly, as three ATPs are required to generate an S -adenosylmethionine molecule, which is then used as methyl donor for cyclopropanation [17] . Therefore, these lipidomic results showed that rpoC mutation promotes energy saving by repressing this costly lipid modification process. The function of cyclopropanation of fatty acid is still not fully understood, although CFAs are known to improve cell resistance to acid stress [17] . In line with reduction in Cfa, a number of other acid resistance proteins (including GadABC, HdeAB and Slp) were also strongly repressed (97–99% reduction) by the rpoC mutation ( Supplementary Fig. 6 ). This result is also consistent with previous studies showing downregulation of acid resistance genes in the RPOC strain [11] , [18] . In addition, stationary phase and stress-induced proteins including Dps, MscS, OsmE, OsmY and Sra were also lowered by 64–81% in RPOC and DKI strains. Interestingly, the level of the ppGpp alarmone was reduced in both RPOC and DKI strains, although the difference was not statistically significant. Collectively, these results suggest that the rpoC mutation relieves E. coli from stress and stationary phase-induced responses during growth on glycerol and allows redeployment of metabolic resources to increase biomass yield. However, the stress response regulator, RpoS, was found to be elevated in RPOC strain, although the level of RpoD was also higher in both RPOC and DKI strains. The increased RpoS level might be related to the fivefold increase in cellular putrescine concentration in the RPOC strain ( Fig. 2a ) [19] , [20] . While the exact molecular mechanism remains to be elucidated, it is possible that this specific rpoC mutation affects its interactions with the sigma factors rpoD and rpoS , thus affecting the stress response. A prior study has shown that some rpoC mutations can vastly modify gene expression particularly those related to motility and acid resistance [11] . Analysis of exo-metabolome showed significantly decreased secretion of N -acetyl aspartate and pyrimidine pathway intermediates (including carbamoylaspartate, dihydroorotate and orotate), in both RPOC and DKI strains compared with the WT and GLPK strains ( Fig. 2e ). Secretion of these metabolites by E. coli has been reported before [21] and the pyrimidines biosynthetic intermediates are known to accumulate in E. coli K-12 because of a mutation in the rph / pyrE [21] , [22] . These observed changes in the exo-metabolome correlate well with the reduction of intracellular concentrations of the same metabolites ( Fig. 2a ), as well as the reduced level of enzymes (PyrBCI) involved in pyrimidine biosynthesis pathway ( Fig. 2f and Supplementary Fig. 6 ). Contrarily to what might be expected, the PyrE protein was not detected in any strain suggesting that the reduced accumulation was not likely due to increased enzyme expression level, in agreement with an earlier study [11] . The fact that pyrimidine intermediates are not secreted in large amounts in RPOC strain and that several enzymes required for their biosynthesis are actually downregulated suggests that either pyrimidine biosynthesis is not a bottleneck for fast growth or that PyrE enzyme activity is regulated by other means that do not involve increased expression. Moreover, the fact that the other enzymes (PyrBCI) known to be negatively regulated by the end products of the pathway are reduced in RPOC suggests there are enough pyrimidines to meet growth needs and also contributes to limit less efficient secretion of intermediates. It is interesting to note that the decrease in these intermediates is even more pronounced in DKI than RPOC strain (epistasis), a difference that may be linked to the faster growth of DKI. Together, the above results indicate that rpoC mutation reprograms E. coli for improved biomass yield by repressing the accumulation of metabolites and energy-wasting processes such as post-synthetic lipid modification, stress and stationary phase-induced responses, and carbon-spilling reactions and secretion ( Fig. 2f ). Interestingly, these are systemic and coordinated responses resulting from a single mutation showing that it acts through multiple mechanisms, as others have reported [2] , [23] . The glpK mutation improves glycerol utilization While the rpoC mutation switches E. coli into carbon saving and high-efficiency mode, the glycerol utilization pattern of the glpK mutant strain suggests that this mutation promotes increased cell growth through a different mechanism. This metabolic difference is evident by a higher secretion of acetate for both the GLPK and DKI strains ( Fig. 3a ). Acetate production and secretion is an overflow mechanism generally interpreted as resulting from an imbalance between carbon uptake/availability and the metabolic network capacity to use it for energy and biomass production [24] . On the other hand, it is also an important source of energy generation through substrate-level phosphorylation [25] . In addition to acetate secretion, we found that both GLPK and DKI strains also secrete significant levels of D -lactate ( Fig. 3b ), succinate and pyruvate ( Fig. 3c ). This elevated level of mixed acid production suggests that the higher glycerol uptake rate induced by the glpK mutation exceeds the need or capacity of cellular metabolism to use the increased carbon flow for biomass formation. Notably, D -lactate production is particularly high in the DKI strain, which could be due to a combined effect of high carbon flow and the elevated ratio of NADH/NAD + cofactor ( Fig. 2c ). Overall, 23% of consumed glycerol was converted to acetate and lactate in DKI strain, followed by GLPK (20%), RPOC (16%) and finally WT (15%). 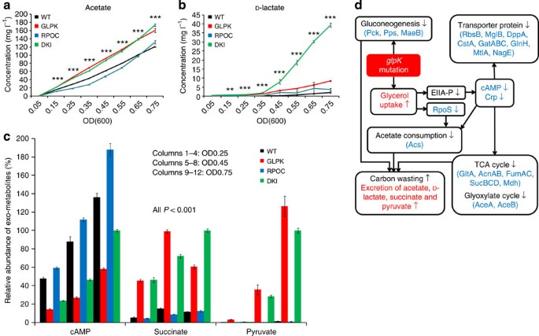Figure 3: Metabolic changes associated with theglpKmutation lead to increased overflow metabolism. (a) Increased secretion of acetate and, (b),D-lactate or (c) cAMP, succinate and pyruvate. Plots show the mean±s.e.Pvalues were obtained from two-way analysis of variance (**P<0.01, ***P<0.001,n=6 foraandb, andn=18 forc). (d) Proposed mechanism of theglpKmutation metabolic effects based on proteomics and metabolomics data. All values incare calculated relative to levels in DKI at OD of 0.75 (100%). Figure 3: Metabolic changes associated with the glpK mutation lead to increased overflow metabolism. ( a ) Increased secretion of acetate and, ( b ), D -lactate or ( c ) cAMP, succinate and pyruvate. Plots show the mean±s.e. P values were obtained from two-way analysis of variance (** P <0.01, *** P <0.001, n =6 for a and b , and n =18 for c ). ( d ) Proposed mechanism of the glpK mutation metabolic effects based on proteomics and metabolomics data. All values in c are calculated relative to levels in DKI at OD of 0.75 (100%). Full size image The type of carbon overflow observed here ( Fig. 3d ) is consistent with a previous study [26] that associated overflow with catabolite repression on glucose and decreased concentrations of acetyl-CoA synthetase and cyclic AMP (cAMP). In the present study, acetyl-CoA synthetase, the key protein for acetate utilization, was markedly repressed (93% reduction) in both GLPK and DKI strains. In addition, cAMP level in the extracellular medium was significantly lowered by the presence of the glpK mutation ( Fig. 3c ). A previous study showed reduced intracellular cAMP level in the GLPK strain, and this result was consistent in three other knock-in strains with different adaptive glpK mutations [10] . This observation is further supported at the proteome level by a twofold decrease of cAMP receptor protein (Crp) in GLPK and DKI strains ( Supplementary Fig. 6 ). In WT E. coli , cAMP-Crp levels are higher during growth on glycerol compared with growth on glucose [27] . Since cAMP-Crp activates tricarboxylic acid (TCA) cycle genes, acetate formation is limited on glycerol, a normally non-fermentable carbon source. On the other hand, the glycerol uptake rate was enhanced in the glpK mutant most probably because of reduced inhibitory effect of fructose 1,6-bisphosphate on GlpK, as shown previously for this mutant [10] . This results in increased transfer of phosphate from phosphorylated EIIA Glc to produce glycerol-3-phosphate [28] . The resulting decrease in phosphorylated EIIA Glc will in turn reduce adenylate cyclase activity and cAMP production. This can then result in repression of the TCA cycle activity, a claim supported by the decreased levels of several enzymes of the TCA cycle (GltA, AcnAB, FumAC, SucBCD and Mdh), the glyoxylate shunt (AceA and AceB) and gluconeogenesis (Pck, Pps and MaeB). Together, these effects result in overflow metabolism and production of acetate, pyruvate and lactate. In addition, the accumulation of pyrimidine pathway intermediates (carbamoylaspartate, orotate and dihydroorotate) also represents a form of overflow metabolism [21] , although the findings in RPOC suggest that it may not be optimal. The decrease in cAMP-Crp is also reflected in the downregulation of transporters, such as MglB (galactose), RbsB (ribose), CstA (peptides), DppA (dipeptides), GatABC (galactitol), GlnH (glutamine), MtlA (mannitol) and NagE ( N -acetylglucosamine; Supplementary Fig. 6 ). The decrease in cAMP levels in glpK mutation containing strains therefore appears responsible for converting glycerol into the observed overflow metabolites. Another interesting possibility is that the glpK mutation, by affecting cAMP levels, may contribute to better optimizing proteomic resources to metabolic needs, as recently proposed [29] . This would suggest that these needs are poorly adjusted in WT E. coli resulting in slower than expected growth. On the basis of these results, we postulate that the decreased cAMP levels and increased glycerol utilization and overflow that are induced by the glpK mutation together result in the increase in growth rate. We note that these changes were not observed in the RPOC strain that displays an intermediate growth rate between the GLPK and DKI strains. The increased carbon flow is probably due to the improved kinetics of mutant GlpK, as well as reduced inhibition by fructose 1,6-bisphosphate, although the level of GlpK actually decreases in the GLPK strain ( Supplementary Table 1 ) [10] . Reduced GlpK expression may appear as a counterintuitive response but it has previously been suggested to be linked to catabolite repression of glpFKX operon owing to reduced cAMP levels and suggested to be important to limit methylglyoxal toxicity [10] . Taken together, glpK mutation appears to promote cell growth by increasing glycerol uptake to a level that may surpass demand and capacity of cell metabolism, leading to increased wasteful carbon overflow. Prior studies have suggested that less efficient overflow metabolism may be advantageous when carbon source is non-limiting and protect against methylglyoxal toxicity [30] . Overflow has also been proposed to represent a trade-off between energy and biomass yield and the biosynthetic costs of respiration that occur during fast growth [31] . In addition, competition for membrane space between substrate uptake and respiration has also been proposed to be a constraint leading to carbon wasting [32] . Our results suggest that the GLPK and RPOC strains may preferentially use overflow/fermentation and respiration, respectively, while the DKI has optimized the balance between these processes and biomass yield to achieve a maximum growth rate. These results agree well with known trade-offs between yield and growth rate during the evolutionary process [33] , [34] . Epistatic effects of rpoC and glpK mutations Mutations in glpK and RNA polymerase ( rpoB / C ) genes were repeatedly found in the glycerol-evolved E. coli strains [8] , suggesting a possible interaction between these two mutations in conferring fitness and growth advantage. On the basis of the results, we postulate that the rpoC mutation may improve growth rate by triggering a carbon-saving response that limits non-essential metabolic activities for optimal glycerol utilization and biomass yield. In such a carbon-saving mode, the bottleneck for biomass production then becomes the glycerol uptake and utilization rate, which is overcome by a mutation in the glpK gene. The combined contribution of rpoC and glpK mutations on growth rate of the DKI strain is about 10% greater than the sum of their individual effects showing that the mutations are epistatic ( Fig. 4 ). The DKI strain may also have improved capacity to counter methylglyoxal toxicity as shown in its more balanced redox state ( Supplementary Fig. 5 ) and the reduced expression of several enzymes involved in methylglyoxal detoxification (AldA, Dld and HchA, and DkgA; Supplementary Table 1 ). 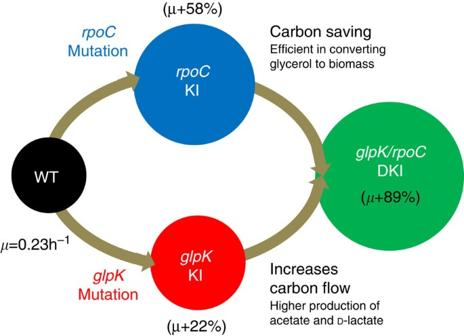Figure 4: Proposed mechanism of action of adaptive mutations inrpoCandglpKon the metabolic phenotype. Whereas therpoCmutation triggers a carbon-saving metabolic state favouring optimal glycerol utilization, mutation in theglpKgene confers a growth advantage by increasing glycerol uptake with concomitant increased carbon wasting. The metabolic contribution of bothrpoCandglpKmutations appear epistatic with combined mutations resulting in a greater growth rate increase than the sum of the effect of both mutations individually. Figure 4: Proposed mechanism of action of adaptive mutations in rpoC and glpK on the metabolic phenotype. Whereas the rpoC mutation triggers a carbon-saving metabolic state favouring optimal glycerol utilization, mutation in the glpK gene confers a growth advantage by increasing glycerol uptake with concomitant increased carbon wasting. The metabolic contribution of both rpoC and glpK mutations appear epistatic with combined mutations resulting in a greater growth rate increase than the sum of the effect of both mutations individually. Full size image The polyomic data revealed that the two mutations in the DKI strain display epistasis that is observable at the metabolic level. The reductions in transporter levels, TCA cycle and glyoxylate enzymes can be linked to the glpK mutation, whereas reductions in the level of stress-related and acid resistance enzymes are triggered by the rpoC mutation ( Supplementary Fig. 6 ). Moreover, the metabolite and proteome profiles of the DKI strain also display unique properties distinct from both GLPK and RPOC strains. Notably, lactate secretion is particularly enhanced (>19-fold, compared with WT) in the DKI strain, and is most apparent at the later phase of growth ( Fig. 3d ). This unique metabolic change shows a synergistic effect of rpoC and glpK mutations, whereby the high NADH/NAD + ratio in the RPOC strain seems to favour conversion of pyruvate to lactate (twofold increase in lactate secretion), while high carbon flow induced by glpK mutation increased its secretion fourfold ( Figs 2c and 3b and Supplementary Fig. 5 ). The enhanced lactate production can regenerate NAD + from NADH (thus, lower NADH/NAD + ratio in Fig. 2c ) to support high glycolytic activity and faster growth in DKI strain. In addition, some other metabolites also seem specifically secreted at higher levels by the DKI strain ( Supplementary Fig. 8 ). In the RPOC strain, the cellular level of putrescine (a polyamine) was increased fivefold as compared with WT ( t -test, Bonferroni-corrected P <0.01, n =6, Fig. 2a ). In E. coli , this polyamine is essential for cell proliferation and normal cell growth [35] , but it was also shown to have negative effects on cell growth at high concentration [36] . Previously, putrescine was also reported to stimulate production of adenylate cyclase and RpoS [19] , [20] . This activation is consistent with the current finding in which both cAMP ( Fig. 2a ) and RpoS ( Supplementary Fig. 4 ) were also increased in the RPOC strain. With the additional mutation in the glpK gene, putrescine concentration in DKI strain was reduced to a level comparable to WT ( t -test, Bonferroni-corrected P >0.05, n =6), and this was accompanied by reductions of cAMP ( Fig. 3c ) and RpoS ( Fig. 3d and Supplementary Fig. 6 ). Therefore, the interaction between rpoC and glpK mutations and the putrescine pathway, and consequently with the numerous genes regulated by cAMP and RpoS might also contribute to increased cell growth in DKI strain. Epistatic interaction between the glpK and rpoC mutations is also apparent in the pyrimidine pathway. With a single mutation in rpoC gene, the RPOC strain reduces carbon wasting in the form of carbamoylaspartate, orotate and dihydroorotate ( Fig. 2e ). The changes are reflected in the DKI strain by even greater reductions in extracellular concentration of these metabolites, as well as intracellular pyrimidine pathway enzymes ( Fig. 2e and Supplementary Fig. 6 ), showing that the carbon-conserving mechanism initiated by the rpoC mutation is further enhanced by glpK mutation in the DKI strain. Together, these features of the DKI strain support and provide specific molecular details for an epistatic effect of the adaptive mutations, leading to enhanced cell growth compared with the combined effect of individual rpoC and glpK mutations. As observed previously, the glpK mutation is a specialist mutation improving growth solely on glycerol, while the rpoC mutation is a generalist one improving growth on several carbon sources [10] , [11] . Our study provides clear mechanistic support in the form of a general energy saving and efficient reorganization of metabolism by rpoC mutation that can improve growth on most carbon sources (on minimal medium) while the effects of glpK mutation are obviously glycerol dependent. The rpoC mutation improved metabolic efficiency and biomass yield, while the fast glycerol utilization following glpK mutation results in faster but more wasteful metabolic function. Together, the DKI combines high biomass yield and metabolic efficiency with fast carbon flow and consequent lactate production to dominate the adaptive evolution landscape on glycerol. While we cannot make direct claims about the universality of our findings (based on the characterization of a single pair of rpoC / glpK mutants) to other mutations in rpoC and glpK that emerge during the evolutionary process, there are good reasons to believe that the findings have greater relevance. First, several different rpoC mutations have been found to generate well-conserved transcriptome changes [11] . In addition, the effects on the pyrimidine biosynthesis pathway appear connected to mutations in rph - pyrE that also contribute to an increase in growth rate when combined with other mutations [8] . This suggests that a metabolic solution to the pyrimidine intermediate accumulation is an important step in increasing growth potential and is not only limited to the mutations we studied here. Moreover, several different glpK mutations have been shown to result in a decrease in cAMP [10] , as observed here, and many of the changes in the metabolome and proteome observed here can be directly connected to cAMP-Crp regulation. Using polyomic data sets (metabolomic, proteomic and lipidomic) obtained from strains harbouring single and combined mutations that improve growth rate of E. coli on glycerol, we have identified two separate but complementary mechanisms for optimizing cellular growth. One mechanism increases biomass yield through reduction in non-essential pathways and improved utilization of carbon while the other improves carbon flow. Both mechanisms together produce global changes that reorganize that metabolic network for optimal growth. The use of energy inefficient and wasteful metabolite overflow appears to be an essential trade-off to achieve fast growth under conditions where carbon source is abundant, as suggested by other studies [31] , [33] . It will be interesting to see how the optimized network of the fast growing mutants described here fares under nutrient-limiting conditions where biosynthetic and efficiency requirements and priorities are different. Our findings bear interesting similarities with two recent related studies about metabolic effects of adaptive evolution of yeast for optimizing growth on galactose [4] , [37] . These authors also uncovered alternative and less intuitive paths leading to growth rate improvements. Together, these different studies demonstrate the importance and power of combining adaptive evolution experiments and polyomic analysis to study the regulatory mechanisms underlying improved metabolic and phenotypic performance under defined selection pressure. They can also provide novel strategies for evolution-based bioengineering applications. E. coli strains and culture All E. coli strains used in the current study were derived from K-12 MG1655 (ATCC 47076) strain. The wild type E. coli refers to genetically unmodified MG1655 (ATCC 47076) stock strain. Two single knock-in strains (GLPK, glpK 218a>t; RPOC, rpoC 27 bp del), as well as a double knock-in strain (DKI, glpK 218a>t+ rpoC 27 bp del; a reconstruction strain of a glycerol-evolved clone) were derived in a previous study [8] and correspond to WT (BOP27) MG1655 ATCC #47076, RPOC (BOP135), GLPK (BOP21)* and DKI (BOP133)*. Before publication, it has come to our attention that while the WT and RPOC strains’ background genotype corresponds to that of E. coli MG1655 ATCC #47076, GLPK* and DKI* strains used in the current study contain three additional non-adaptive mutations (that is, btuE , hisC and ydaC ), as they were originally inserted in WT-A background [8] . Although this does not affect the interpretation of the effects of the rpoC mutation, it is a potentially confounding factor in studying the effect of glpK mutation. Nevertheless, a previous study showed that these mutations do not confer any growth advantage or affect the growth rate of E. coli on glycerol minimum media [8] . Furthermore, the core metabolic changes found in GLPK and DKI strain, including the observed decrease in cAMP and catabolite repression are known to be directly caused by glpK mutation, and have been repeatedly observed in a number of glpK mutants, with and without the non-adaptive mutations [10] . In addition, glpK mutation effects (as shown in Fig. 3d ), including changes in transporter proteins, gluconeogenesis, TCA cycle, glyoxylate cycle, acetate consumption and carbon-wasting mechanism have previously been similarly associated with decreased levels of cAMP, catabolite repression and increased growth rate in E. coli [21] , [26] . Moreover, most changes observed in the RPOC strain (containing no additional non-adaptive mutations) are overall dominant and well reflected in the DKI strain ( Fig. 2a and Supplementary Figs 3 and 4 ), supporting that their origin is specific to rpoC mutation. Therefore, there is very strong support to conclude that the current findings observed in GLPK and DKI strains can be attributed specifically to the adaptive glpK mutation and the combination of glpK and rpoC mutation, respectively. Main cultures ( n =6) were grown in 185 ml of M9 minimal medium with 2 g l −1 of glycerol as carbon source in 500 ml Erlenmeyer flasks, incubated at 30 °C in a water bath and aerated by magnetic stirring bars spinning at 1,000 r.p.m. This number of replicate was chosen to optimize the power of the study while considering available resources. Sample preparation At OD 600 from 0.05 to 0.75 (0.1 OD intervals), 1.5 ml samples were filtered through a 0.2-μm cellulose acetate syringe filter, and the filtrates were stored at −80 °C before exo-metabolome analysis. At OD 600 of 0.25, 0.45 and 0.75, samples were collected (sampling volume in ml, V =20/OD 600 ) for metabolomics, proteomics and lipidomics analysis. In brief, cells were filtered by a vacuum filtration system using a 0.4-μm pore size filter, and metabolites and lipids were extracted using a methanol–chloroform–water extraction method [38] . The methanol used contained 5 μM each of methionine sulphone and D -camphor-10-sulphonic acid as internal standards for metabolomics. In addition, two internal standards for lipidomics (10 μM each of 1,2-dimyristoyl(d54)-sn-glycero-3-phosphocholine and 1,2-dihexanoyl(d22)-sn-glycero-3-phosphocholine) were added in the chloroform used in the extraction process. Glassware was used throughout the lipid extraction process to prevent contamination from plastic extractives. Note that some of the experiments display data for cell samples at optical densities of 0.25, 0.45 and 0.75, while most emphasize only 0.25. This choice is based on the fact that adaptive evolution was performed on cells that were kept at the early- to mid-exponential stage for the whole duration of the process [3] . In this case, we can therefore expect that the evolutionary process may result in a response that is optimized for lower cell density conditions. For this reason, our main conclusions emphasize findings for cells at 0.25, mainly to be consistent with the conditions under which adaptive evolution was conducted. However, the data collected at later time points are also relevant and, especially for the exo-metabolome, the higher cell densities thereof, make it easier to detect secreted metabolites. Most endo-metabolome changes are consistent for all three sampling points. Metabolomics Dried aqueous metabolites were reconstituted with 50 μl of Milli-Q water that contained two reference compounds (200 μM each of 3-aminopyrrolidine and trimesic acid). Samples were analysed using capillary electrophoresis-electrospray ionization (ESI)–time-of-flight mass spectrometry (TOFMS) in both positive and negative mode [39] . In brief, cationic metabolites were separated in a fused silica capillary (50 μm i.d. × 100 cm total length) filled with 1 mol l −1 formic acid as the reference electrolyte. The sheath liquid was methanol/water (50% v/v) containing 0.1 μmol l −1 Hexakis and was delivered at 10 μl min −1 . ESI–TOFMS was operated in positive-ion mode, and mass spectra were acquired at a rate of 1.5 cycles per second from m / z 50 to 1,000. In addition, anionic metabolites were separated in a commercially available COSMO(+) capillary, which was chemically coated with a cationic polymer. Ammonium acetate solution (50 mmol l −1 , pH 8.5) was used as the electrolyte for capillary electrophoresis separation. Ammonium acetate (5 mmol l −1 ) in methanol/water (50% v/v) containing 0.1 μmol l −1 Hexakis was delivered as the sheath liquid at 10 μl min −1 . ESI–TOFMS was operated in negative-ion mode and mass spectra were acquired at a rate of 1.5 cycles per second from m / z 50 to 1,000. The obtained data were processed using in-house software (MasterHands) [40] . The data set is available in Supplementary Data 1 . Proteomics The protease inhibitor, 4-(2-aminoethyl)benzenesulphonyl fluoride hydrochloride was added to 100 μl cell lysate (final concentration of 1 mmol l −1 ), and the samples were stored in −80°C freezer until further analysis. Proteins were extracted with 12 mmol l −1 sodium deoxycholate, 12 mmol l −1 sodium N -lauroylsarcosinate and 100 mmol l −1 Tris–HCl (pH 9.0), reduced with 10 mmol l −1 dithiothreitol at room temperature for 30 min, and alkylated with 50 mmol l −1 iodoacetamide in the dark at room temperature for 30 min. The protein mixture was diluted fivefold with 50 mmol l −1 ammonium bicarbonate, digested with Lys-C, followed by trypsin digestion overnight. An equal volume of ethyl acetate was added to the sample solution and the mixture was acidified with 0.5% trifluoroacetic acid (final concentration) according to the phase-transfer surfactants protocol [41] . In brief, the mixture was shaken for 1 min and centrifuged at 15,700 g for 2 min, and then the aqueous phase was collected. Peptides were desalted using C18-StageTips [42] , [43] , [44] , and labelled with isotopomeric dimethyl labels [45] . In brief, peptides were dissolved with 100 mmol l −1 triethyl ammonium bicarbonate and labelled with formaldehyde and cyanoborohydride for 60 min. In the current study, a pooled sample from all studied strains was labelled with CH 2 O (light), while each sample was labelled with 13 CD 2 O (heavy). The reaction was terminated by adding ammonium solution, and then mixed together before the desalting step using C18-StageTip. Then, the samples were analysed using an LTQ-Orbitrap XL (Thermo Fisher Scientific, Bremen, Germany) with a nanoLC interface (Nikkyo Technos, Tokyo, Japan) [46] . The acquired raw data files were analysed by Mass Navigator v1.2 (Mitsui Knowledge Industry, Tokyo, Japan) to create peak lists on the basis of the recorded fragmentation spectra for Mascot v2.2 (Matrix Science, London) and using, for identification, E. coli K-12 proteins registered in GenoBase (4,316 entries, as of 31 January 2006, http://www.ecoli.naist.jp/GB8-dev/index.jsp?page=genome_download.jsp ). A precursor mass tolerance of 3 p.p.m. and a fragment ion mass tolerance of 0.8 Da were employed with strict trypsin specificity, allowing for up to two missed cleavages. Carbamidomethylation of cysteine was set as a fixed modification, while dimethylation of N-termini and primary amino groups of lysine, as well as methionine oxidation, were allowed as variable modifications. Peptides were rejected if the Mascot score was below the 95% confidence limit based on the ‘identity’ score of each peptide, and a minimum of two peptides with at least seven amino-acid residues was required for protein identification. In cases where the identified protein was a member of a multiprotein family featuring similar sequences, the protein was identified according to the highest number of matched peptides and Mascot score. False-positive rates were estimated by searching against a randomized decoy database created by the Mascot Perl program supplied by Matrix Science. In total, 768 proteins based on 8,349 peptides (false discovery rate: 0.88%) were identified in the proteomic study. The data set is available in Supplementary Data 1 . Lipidomics Lipid extracts were analysed using a liquid chromatography–TOFMS (LC–TOFMS) using an Ascentis Express C8 column (particle size, 2.7 μm; ø 2.1 × 150 mm i.d. ; Sigma-Aldrich, St Louis, MO, USA) [47] . In brief, the mobile phase used was composed of Milli-Q water containing 10 mmol l −1 ammonium acetate (A) and isopropanol (B). The gradient started with a composition of 45% B, which was linearly increased to 99% B over 40 min with holding for 5 min. For each analysis, the mobile phase was pumped at a flow rate of 200 μl min −1 . TOFMS was conducted in the positive-ion mode: the capillary voltage was set at 4 kV; nitrogen gas (350 °C) was used for ESI; the fragmenter, skimmer and octopole radio frequency voltage were set at 250, 60 and 250 V; mass spectra were acquired at the rate of 1.0 cycles s −1 over an m / z range of 50–1,650. Raw data from LC–TOFMS were processed using in-house software (MasterHands) [40] . Relative abundance of lipids was calculated using lipid internal standard. For determination of lipid species and acyl chain length, lipid samples from each E. coli strains were analysed using a LC–MS/MS. In brief, reversed-phase LC separation was achieved by ACQUITY UPLC HSS column (particle size, 1.8 μm, 50 × 2.1 mm i.d., Waters Corporation, Milford, MA, USA) at 45 °C. The mobile phase was prepared by mixing solvents (A) acetonitrile/methanol/water (20/20/60; 5mmol l −1 ammonium formate) and (B) isopropanol (5mmol l −1 ammonium formate). The mobile phase was pumped at a flow rate of 300 μl min −1 . LC–MS/MS analysis was performed using Triple Quad 5500 System (AB SCIEX, Foster City, CA, USA) with an Agilent 1290 Infinity LC system (Agilent Technologies, Loveland, CO, USA) in the negative-ion mode. Each glycerophospholipid was identified by the product ion peaks of fatty acids and polar head group from MS/MS analysis. The data set is available in Supplementary Data 1 . It should be noted that the analytical method used does not allow to distinguish cy17:0 and cy19:0 from their corresponding isobaric unsaturated 17:1 and 19:1 fatty acids. This is a common limitation for most LC–MS and LC–MS/MS-based lipidomic studies that identify lipids based on the product ion signals of fatty acids. However, neither 17:1 nor 19:1 unsaturated fatty acids are known to be produced by E. coli and the observed signals were therefore assigned to CFA, in line with prior studies [14] , [15] , [16] . Exo-metabolome analysis A total of 192 dried samples were reconstituted in 500 μl of 150 mmol l −1 phosphate buffer (including K 2 HPO 4 and NaH 2 PO 4 in D 2 O, pH 7.4) containing 0.58 mmol l −1 sodium-3-(tri-methylsilyl)-2,2,3,3-tetradeuteriopropionate (TSP) as an internal standard and chemical shift standard. The samples were analysed by 1 H-NMR spectroscopy at 499.84 MHz using a Varian 500 MHz NMR spectrometer equipped with a triple resonance probe (Palo Alto, CA, USA) at 293 K, using a solvent suppression pulse sequence based on a one-dimensional nuclear Överhauser enhancement spectroscopy pulse sequence. A total of 64 transients with a spectral width of 10 kHz and 20,000 data points (that is, acquisition time of 2 s) were collected for every NMR spectrum. The NMR spectra were processed using MestRe-C software (version 4.8, http://mestrelab.com/ ). Spectra were Fourier transformed, referenced to TSP at 0.0 p.p.m. and were phase- and baseline-corrected manually. Each spectrum was integrated using 0.005 p.p.m. integral regions between −0.5 and 9.0 p.p.m. The region containing water (4.5–6 p.p.m.) was excluded from further analysis. Each integral region was normalized to the integral value of TSP for each spectrum. All NMR peaks were assigned according to the Human Metabolome database ( http://www.hmdb.ca/ ) [48] , published literature [49] and Chenomx NMR suite version 7.5 (Chenomx, Alberta, Canada). Metabolite concentrations were estimated using Chenomx NMR suite. Enantiomeric determination of D -lactate was confirmed using enzymatic assays (Boehringer Mannheim, R-Biopharm, Darmstadt, Germany). In addition, acetate concentration in the culture medium was also monitored using enzymatic assays (Boehringer Mannheim, R-Biopharm). To widen the coverage of exo-metabolome and complement the NMR data, exo-metabolites collected at OD 600 of 0.25, 0.45 and 0.75 were analysed using LC–TOFMS and LC–MS/MS. First, samples were analysed using a LC–TOFMS to identify metabolites present in the spent culture media. Then, these metabolites were targeted for analysis using a LC–MS/MS operating in multiple reaction monitoring mode. The multiple reaction monitoring parameters for each metabolite were determined using authentic metabolic standards, and optimized using the Optimizer feature of the MassHunter software (Agilent Technologies). LC–MS/MS was carried out using an Agilent 1,200 series HPLC system (Agilent Technologies) and an Agilent 6430 triple quadrupole mass spectrometer. Metabolites separation was carried out on a pentafluorophenylpropyl column (Luna PFP (2), 150 × 2 mm, 3 μm, Phenomenex, Torrance, CA, USA) [50] . In brief, the mobile phase A used was composed of water with 0.1% (v/v) formic acid and mobile phase B was acetonitrile. A linear gradient was used for positive ESI mode with a total run time of 40 min at 0.20 ml min −1 : 0% B (0–8 min), 0–25% B (8–26 min), 25–100% B (26–28 min), 100% B (28–33 min), 100–0% B (33–34 min) and 0% B (34–40 min). In addition, the total run time for negative ESI mode was 34 min at 0.20 ml min −1 , using a linear gradient: 0% B (8 min), 0–30% B (8–15 min), 30–50% B (15–16 min), 50% B (16–21 min), 50–100% B (21–22 min) and 100% B (22–27 min), 100–0% B (27–28 min) and 0% B (28–34 min). The injection volume was 5 μl for both positive and negative modes. System control, data acquisition and analysis were performed using MassHunter software. The data set is available in Supplementary Data 1 . Cell size and number At OD 600 of 0.25, 0.45 and 0.75, cells were sampled and fixed with formaldehyde (0.1% final concentration). The cell density and volume were measured using a particle analyser, CDA-1000 (Sysmex, Japan). As shown in Supplementary Fig. 1a , cell volume is considerably affected by the mutations. This observation agrees with the known increase in cell volume with increase in growth rate but suggests that growth rate is not the only factor since GLPK cells are much smaller than RPOC cells, although they have similar growth rates. Moreover, at higher OD where growth rate should be reduced, RPOC cells retain a large volume. While such differences in cell size could potentially affect concentration measurements, all metabolite levels reported were normalized to unit OD and Supplementary Fig. 1b shows that the total cell volume in all strains varies by <20% from WT and will not significantly affect results or conclusions of our study. Statistical analysis Metabolomics, lipidomics and proteomics data were analysed using t -test and analysis of variance in MATLAB (The MathWorks), and the P values shown were corrected with Bonferroni correction unless otherwise specified. In addition, the metabolomic data set was imported into SIMCA-P+ 11.0 (Umetrics, Umeå, Sweden) for processing using PLS-DA. How to cite this article: Cheng, K.-K. et al. Global metabolic network reorganization by adaptive mutations allows fast growth of Escherichia coli on glycerol. Nat. Commun. 5:3233 doi: 10.1038/ncomms4233 (2014).